Cell transcriptional state alters genomic patterns of DNA double-strand break repair in human astrocytes The misrepair of DNA double-strand breaks in close spatial proximity within the nucleus can result in chromosomal rearrangements that are important in the pathogenesis of haematopoietic and solid malignancies. It is unknown why certain epigenetic states, such as those found in stem or progenitor cells, appear to facilitate neoplastic transformation. Here we show that altering the transcriptional state of human astrocytes alters patterns of DNA damage repair from ionizing radiation at a gene locus-specific and genome-wide level. Astrocytes induced into a reactive state exhibit increased DNA repair, compared with non-reactive cells, in actively transcribed chromatin after irradiation. In mapping these repair sites, we identify misrepair events and repair hotspots that are unique to each state. The precise characterization of genomic regions susceptible to mutation in specific transcriptional states provides new opportunities for addressing clonal evolution in solid cancers, in particular those where double-strand break induction is a cornerstone of clinical intervention. Genomic instability and genetic heterogeneity are key players in clonal evolution and diversification in malignant neoplasms, ultimately leading to the failure of cytotoxic and targeted therapies [1] , [2] , [3] . Although progress has been made in the identification and characterization of important driver mutations, the origin of these and the significance of passenger mutations remain poorly understood. Elucidating the mechanisms and determinants of the genomic instability that gives rise to such mutations will provide an avenue towards new therapeutic approaches that attempt to prevent clonal evolution directly. Several recent studies have revealed the major roles nuclear organization and DNA double-strand breaks (DSBs) play in the pathogenesis of oncogenic chromosomal rearrangements in B-cell precursors, where programmed DSBs underlie immune adaptation [4] , [5] . However, the concept that genomic instability can be mediated by the non-homologous end-joining (NHEJ) of DSBs in close spatial proximity probably applies to a broader range of cell types and their neoplastic counterparts [6] , [7] . Glial progenitor cells are of particular interest, because they give rise to incurable neoplasms (gliomas) with remarkable phenotypic and genetic heterogeneity, as epitomized by glioblastoma multiforme (GBM). The standard first-line treatment for malignant gliomas, including GBM, consists of fractionated radiotherapy and temozolomide [8] , both of which are potent DSB-inducing agents [9] . As nuclear architecture is not random, but highly organized into transcriptionally active and inactive domains [10] , we reasoned that the genomic pattern of DSB repair after exposure to ionizing radiation (IR) would also be non-random and, moreover, influenced by the transcriptional state of the cell. To provide evidence of this interaction, we take advantage of the ability of astrocytes to undergo a transition in transcriptional state in response to a mechanical stimulus [11] . Phenotypically, this state of activation is characterized by elevated expression of intermediate filaments [12] , increased secretion of cytokines and extracellular matrix components [13] , cell hypertrophy [14] , proliferation [15] and migration [16] . Activated astrocytes also express elevated levels of the progenitor marker nestin [17] , [18] , [19] , adopt a bipolar morphology [20] , [21] and can be used to generate neurospheres that are differentiable into neurons and oligodendrocytes [22] , [23] , [24] . Together, these features are suggestive of a more primitive state of differentiation and recapitulate some of the phenotypic attributes of glioma cells [11] , [25] . Using geometric arrangements of scratch-activated and confluent human astrocytes derived from primary cultures, we conduct comparative, correlative analyses to establish a chain of causation between the transcriptional state of the cell and gene locus-specific susceptibility to mutation following IR. We identify loci within two genes, Rb1 and Srgn , which exhibit distinct patterns of IR-induced chromosomal rearrangement in a transcriptional state-dependent manner. Phenotype of scratch-edge cells Normal human astrocytes (NHAs) isolated from cerebral neocortex of second trimester fetuses and histologically normal cortical specimens from adult epilepsy surgery patients were grown to confluence over 6 weeks, passaged once and transferred to coated chamber slides. These cells exhibited a fibrous morphology with long, branched processes ( Supplementary Fig. 1a ). After achieving confluence in 10–14 days, there was low-to-moderate expression of glial fibrillary acidic protein (GFAP) and nestin in a subset of cells, indicating that many cells were in a quiescent differentiated state ( Supplementary Fig. 1b,c ). Nuclear SOX2 expression was largely absent. Twenty-four hours after linearly scratching the monolayers, fetal NHAs at the scratch edge exhibited a bipolar morphology with unbranched processes terminating in conical end feet. These cells intensely expressed GFAP, nestin and SOX2 ( Supplementary Fig. 1d–f ), while the expression pattern away from the scratch edge did not change significantly. Scratch-edge adult NHAs took up to 48 h to exhibit similar changes in morphology and gene expression ( Supplementary Fig. 1g,h ). Taken together, these results indicate that activation by mechanical disruption of contact inhibition induces quiescent NHAs into a state with several phenotypic features of glial progenitor cells. γH2AX foci in scratch-activated NHA nuclei after IR Histone H2A.X is rapidly phosphorylated at serine 139 in response to DNA DSBs by phosphatidylinositide 3-kinase-like kinases [26] , is highly specific and readily detected immunocytochemically [9] . Foci of γH2AX grow in size, peaking at 30 min after injury, and serve to create a platform for DNA response and repair factors on opened chromatin [27] , [28] , [29] . γH2AX is dephosphorylated or removed from the chromatin structure as DNA repair mechanisms cease [30] , [31] . We scratched confluent monolayers of fetal and adult NHAs and then irradiated them with a 5-Gy dose of X-rays 24 and 48 h later, respectively, to allow the majority of scratch-edge cells to transition into the activated state. Nuclei of GFAP-positive, nestin-positive activated NHAs migrating into the scratch wound uniformly exhibited large numbers of γH2AX foci compared with non-activated cells outside the scratch area ( Fig. 1 ). These foci were apparent 30 min after irradiation and returned to baseline levels by 24 h, consistent with dephosphorylation of γH2AX and cessation of DNA repair ( Supplementary Fig. 2a–d ). To rule out γH2AX foci formation simply as a result of scratch injury, non-irradiated scratched monolayers of fetal and adult NHAs were similarly investigated ( Fig. 1a,b ). These cells demonstrated low-level nuclear patterns of foci similar to NHAs in non-irradiated, non-scratched monolayers ( Supplementary Fig. 2e ), and NHAs in non-irradiated, scratched monolayers distant from the scratch edge ( Supplementary Fig. 2f ). Irradiation of confluent monolayers tended to produce patchy clusters of cells showing high levels of γH2AX foci within the nuclei ( Supplementary Fig. 2g ). Nuclear levels of non-phosphorylated H2AX were similar in confluent and scratched NHAs before and after irradiation ( Supplementary Figs 3 and 4 ). The presence and repair of DSBs was confirmed with a second marker, 53BP1 ( Supplementary Fig. 5 ), and the neutral comet assay ( Supplementary Fig. 6 ). 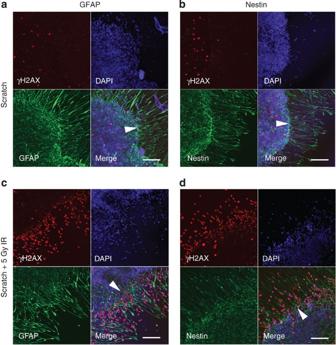Figure 1: Pattern of H2AX phosphorylation in scratched monolayers of fetal NHAs. (a) Fetal NHA monolayers were grown to confluence over 10 days, scratched with a pipette tip and fixed 24 h later. Monolayers were co-stained for GFAP and γH2AX, and counterstained with 4′,6-diamidino-2-phenylindole (DAPI). (b) Same as ina, but monolayers were co-stained for nestin and γH2AX, and counterstained with DAPI. (c) Same as ina, but monolayers were irradiated with 5 Gy X-rays 24 h after scratch and fixed 30 min later. (d) Same as inb, but monolayers were irradiated with 5 Gy X-rays 24 h after scratch and fixed 30 min later. Arrowheads indicate scratch edge and direction of cell migration. Scale bars, 100 μm. Figure 1: Pattern of H2AX phosphorylation in scratched monolayers of fetal NHAs. ( a ) Fetal NHA monolayers were grown to confluence over 10 days, scratched with a pipette tip and fixed 24 h later. Monolayers were co-stained for GFAP and γH2AX, and counterstained with 4′,6-diamidino-2-phenylindole (DAPI). ( b ) Same as in a , but monolayers were co-stained for nestin and γH2AX, and counterstained with DAPI. ( c ) Same as in a , but monolayers were irradiated with 5 Gy X-rays 24 h after scratch and fixed 30 min later. ( d ) Same as in b , but monolayers were irradiated with 5 Gy X-rays 24 h after scratch and fixed 30 min later. Arrowheads indicate scratch edge and direction of cell migration. Scale bars, 100 μm. Full size image In addition, fetal scratch-edge cell nuclei did not preferentially incorporate 5-bromo-2′-deoxyuridine (BrDU) compared with cells distant from the edge, indicating that NHA activation was not simultaneously accompanied by an increase in DNA content ( Supplementary Fig. 7 ). Thus, the higher levels of γH2AX foci in the nuclei of scratch-activated cells compared with inactivated cells after IR cannot be accounted for either by DSBs caused by direct nuclear trauma or spontaneous DSBs occurring during DNA replication. γH2AX foci form preferentially in euchromatin γH2AX nuclear foci have been shown to co-localize with actively transcribing euchromatic regions in a variety of cell types, suggesting that more compact heterochromatic regions may be resistant to H2AX phosphorylation [32] , [33] , [34] . To elucidate the relationship between chromatin state and DSB repair in NHAs, irradiated scratch-edge fetal NHAs were co-stained with antibodies against γH2AX and either di-/trimethyl-lysine-4-histone H3 (H3K4Me2/3) to detect euchromatin, or di-/trimethyl-lysine-9-histone H3 (H3K9Me2/3) to detect heterochromatin [35] . Nuclei were counterstained with 4′,6-diamidino-2-phenylindole, which preferentially stains heterochromatin ( Fig. 2a,b ). 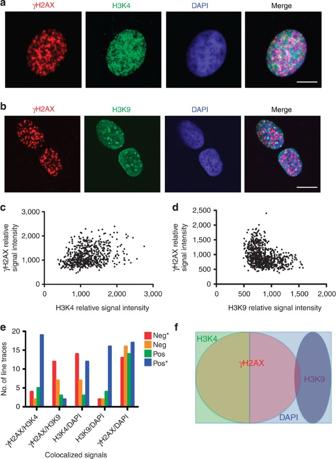Figure 2: γH2AX foci in scratch-activated NHAs occur preferentially in euchromatin. (a) Nuclei of fetal NHAs migrating into scratch defects were co-stained with antibodies against γH2AX (green) and di-/trimethyl-lysine-4-histone H3 (H3K4, red), and counterstained with 4’,6-diamidino-2-phenylindole (DAPI; blue). (b) Same as ina, but nuclei were co-stained for γH2AX (red) and di-/trimethyl-lysine-9-histone H3 (H3K9, green), and counterstained with DAPI (blue). (c) Representative plot correlating γH2AX and H3K4 immunofluorescence relative signal intensities along a line trace through a single scratched-cell nucleus containing 413 data points. Spearmanr=0.3413,P<0.0001. (d) Same as inc, except γH2AX and H3K9 signals are correlated along a line trace containing 831 data points. Spearmanr=−0.3356,P<0.0001. (e) Graph showing distribution of correlation coefficients among line traces (data sets). Correlation coefficients are categorized as significantly negative (red,r<0,P<0.05), non-significantly negative (orange,r<0,P>0.05), non-significantly positive (green,r>0,P>0.05), or significantly positive (blue,r>0,P<0.05). (f) Schematic, based one, illustrating spatial relationships between analysed signals within the nucleus. Scale bars, 10 μm.Pvalues were calculated using the two-tailed Student’sttest. Figure 2: γH2AX foci in scratch-activated NHAs occur preferentially in euchromatin. ( a ) Nuclei of fetal NHAs migrating into scratch defects were co-stained with antibodies against γH2AX (green) and di-/trimethyl-lysine-4-histone H3 (H3K4, red), and counterstained with 4’,6-diamidino-2-phenylindole (DAPI; blue). ( b ) Same as in a , but nuclei were co-stained for γH2AX (red) and di-/trimethyl-lysine-9-histone H3 (H3K9, green), and counterstained with DAPI (blue). ( c ) Representative plot correlating γH2AX and H3K4 immunofluorescence relative signal intensities along a line trace through a single scratched-cell nucleus containing 413 data points. Spearman r =0.3413, P <0.0001. ( d ) Same as in c , except γH2AX and H3K9 signals are correlated along a line trace containing 831 data points. Spearman r =−0.3356, P <0.0001. ( e ) Graph showing distribution of correlation coefficients among line traces (data sets). Correlation coefficients are categorized as significantly negative (red, r <0, P <0.05), non-significantly negative (orange, r <0, P >0.05), non-significantly positive (green, r >0, P >0.05), or significantly positive (blue, r >0, P <0.05). ( f ) Schematic, based on e , illustrating spatial relationships between analysed signals within the nucleus. Scale bars, 10 μm. P values were calculated using the two-tailed Student’s t test. Full size image Confocal microscopy of co-stained scratch-edge NHA nuclei was used to correlate the relative immunofluorescence signal intensities of the two antibodies along line traces containing at least 400 points for a single nucleus ( Fig. 2c,d and Supplementary Figs 8–10 ). The degree of correlation of each pair of antibodies in at least 25 cell nuclei was ascertained ( Fig. 2e ). Based on these co-localization results, we constructed a schematic illustrating overall staining relationships within the nuclear compartment ( Fig. 2f ). Notably, γH2AX and H3K9Me2/3 stained mutually exclusive compartments, while there was significant co-localization of γH2AX and H3K4Me2/3. Adult NHAs exhibited similar co-localization relationships. To further assess the relationship between genomic regions undergoing active transcription and the formation of γH2AX foci, we treated scratched NHAs with α-amanitin, an inhibitor of RNA polymerase II and III, for 24 h before exposure to IR ( Supplementary Fig. 11a ). Increasing concentrations of α-amanitin were associated with lower levels of γH2AX in scratched NHAs as detected by immunoblotting. In confluent NHAs, pretreatment with α-amanitin conversely tended to increase levels of γH2AX. Furthermore, in a separate experiment where NHAs were irradiated at increasing time intervals after scratch, cells formed the greatest number of γH2AX foci 24 to 48 h after scratch ( Supplementary Fig. 11b ). Levels of γH2AX foci after irradiation 72–96 h after scratch were similar to levels in irradiated confluent cells. Together, these results indicate that γH2AX foci preferentially develop in euchromatic domains within the nuclei of scratch-activated NHAs exposed to IR, and that this effect can be reversed by transcriptional blockade or by allowing cells to return spontaneously to a relatively quiescent state. Regions of constitutive heterochromatin and transcriptional silencing tended not to develop γH2AX foci. Scratch activation heightens DSB repair in fetal NHAs To investigate the effects of scratch activation and IR on the proliferation potential of NHAs, fetal and adult NHAs at passage 1 were grown to confluence and scratched. When the majority of cells along the scratch edge had acquired the activated phenotype, we administered a 5-Gy fraction of X-rays. Cells were then transferred into tissue culture flasks and serially passaged in low-serum NHA medium until senescence ( Fig. 3 ). 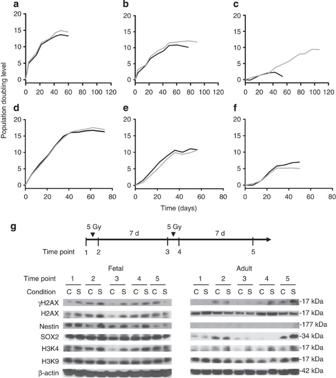Figure 3: Change in PDL of confluent and scratched NHAs over time. (a) Fetal NHAs were grown to confluence in plates, scratched (grey curve) or left unscratched (black curve) at 0 h, transferred to flasks at 72 h and serially passaged until senescence. Time indicated is from transfer to flask. (b) Same as ina, except 5 Gy of X-rays was administered to cells at 24 h. (c) Same as inb, except cells underwent a second round of scratch (or sham scratch) followed by 5 Gy irradiation at 7 and 8 days, respectively, before being transferred to flasks at 10 days. The experiment was performed in duplicate. (d–f) Same as ina–c, except adult NHAs were used. (g) Western blotting showing expression levels of indicated proteins in confluent (C) and scratched (S) fetal and adult NHAs during radiation time course used ina–f. Time points indicated are: (1) before 5 Gy IR; (2) 30 min following 5 Gy IR; (3) before second 5 Gy dose (7 days later); (4) 30 min following second 5 Gy dose; (5) 7 days following second 5 Gy dose. Figure 3: Change in PDL of confluent and scratched NHAs over time. ( a ) Fetal NHAs were grown to confluence in plates, scratched (grey curve) or left unscratched (black curve) at 0 h, transferred to flasks at 72 h and serially passaged until senescence. Time indicated is from transfer to flask. ( b ) Same as in a , except 5 Gy of X-rays was administered to cells at 24 h. ( c ) Same as in b , except cells underwent a second round of scratch (or sham scratch) followed by 5 Gy irradiation at 7 and 8 days, respectively, before being transferred to flasks at 10 days. The experiment was performed in duplicate. ( d – f ) Same as in a – c , except adult NHAs were used. ( g ) Western blotting showing expression levels of indicated proteins in confluent (C) and scratched (S) fetal and adult NHAs during radiation time course used in a – f . Time points indicated are: (1) before 5 Gy IR; (2) 30 min following 5 Gy IR; (3) before second 5 Gy dose (7 days later); (4) 30 min following second 5 Gy dose; (5) 7 days following second 5 Gy dose. Full size image Non-irradiated, non-scratched fetal and adult NHAs achieved maximum population doubling levels (PDLs) of 13.67 and 16.74, respectively ( Fig. 3a,d , black curves). For both cell types, non-irradiated, scratched cells achieved slightly higher PDLs of 14.93 and 17.58, respectively ( Fig. 3a,d , grey curves). Singly and doubly irradiated adult NHAs, whether scratched or not, achieved successively lower PDLs ( Fig. 3e,f ). Interestingly, although scratched and unscratched singly irradiated fetal NHAs achieved similar PDLs, doubly scratched and irradiated fetal NHAs achieved a far higher PDL (9.43) compared with fetal NHAs that had received a similar dose of radiation, but had not been scratched before irradiation (2.29). A similar effect of scratch on proliferation rate, unique to doubly but not singly treated monolayers, was observed in a primary culture of simian astrocytes ( Supplementary Fig. 12 ). Fetal and adult NHAs that were subjected to three or more rounds of irradiation, scratched or not, did not proliferate. Western blot analysis of fetal and adult NHAs during the two rounds of irradiation demonstrated high levels of γH2AX 1 week following the second fraction of X-rays in all conditions, except scratched fetal NHAs ( Fig. 3g and Supplementary Figs 13 and 14 ). Thus, scratched fetal NHAs retained their capacity to repair IR-induced DSBs, while cells in the other conditions continued to exhibit evidence of extensive DNA damage. Taken together, these results suggest that the elevated levels of γH2AX observed in the nuclei of scratch-activated compared with confluent fetal NHAs 30 min after irradiation correspond to higher levels of DNA repair. This was associated with higher rates of cell proliferation, achieved PDL and thus a relative gain in cellular fitness. Activation alters DSB repair levels at selected gene loci To test whether repair of IR-induced DSBs occurs differentially at specific genetic loci in scratched and confluent fetal NHAs, we precipitated cross-linked digested chromatin using anti-γH2AX antibodies and compared the relative enrichment of selected loci using quantitative PCR (qPCR). Western blot analysis confirmed efficient immunoprecipitation and overall higher levels of γH2AX in scratched compared with confluent fetal NHAs after irradiation, despite the presence of fewer numbers of cells due to scratch defects ( Fig. 4a ). 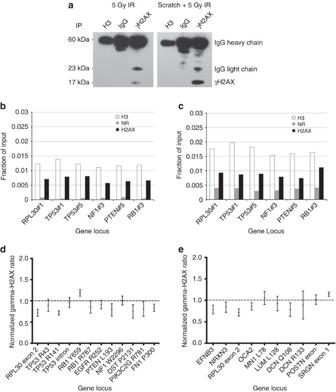Figure 4: ChIP-qPCR analysis of confluent and scratched fetal NHAs. (a) Cross-linked chromatin from confluent or scratched monolayers of fetal NHAs was immunoprecipitated using normal rabbit IgG, or antibodies against histone H3 or γH2AX, resolved using SDS–PAGE and immunoblotted for γH2AX. (b) Representative qPCR analysis of six gene loci using chromatin from irradiated confluent fetal NHAs. SeeSupplementary Table 2for primers used. (c) Same as inb, except chromatin from irradiated scratched fetal NHAs was used. (d) Mean scratch-to-confluent ratio of normalized γH2AX qPCR signals for loci exhibiting high rates of somatic mutation in GBM. Bars are s.e. for four biological replicates, with each replicate consisting of the average of technical duplicates. (e) Same as indfor loci overexpressed in scratched compared with confluent fetal NHAs. Figure 4: ChIP-qPCR analysis of confluent and scratched fetal NHAs. ( a ) Cross-linked chromatin from confluent or scratched monolayers of fetal NHAs was immunoprecipitated using normal rabbit IgG, or antibodies against histone H3 or γH2AX, resolved using SDS–PAGE and immunoblotted for γH2AX. ( b ) Representative qPCR analysis of six gene loci using chromatin from irradiated confluent fetal NHAs. See Supplementary Table 2 for primers used. ( c ) Same as in b , except chromatin from irradiated scratched fetal NHAs was used. ( d ) Mean scratch-to-confluent ratio of normalized γH2AX qPCR signals for loci exhibiting high rates of somatic mutation in GBM. Bars are s.e. for four biological replicates, with each replicate consisting of the average of technical duplicates. ( e ) Same as in d for loci overexpressed in scratched compared with confluent fetal NHAs. Full size image We selected eight loci known to be mutated at a high rate in GBM samples based on Cancer Genome Atlas and COSMIC data [36] . As our data indicated the preferential accumulation of γH2AX within euchromatin, we selected an additional eight loci based on genes that demonstrated >2-fold differential expression in scratched compared with confluent fetal NHAs ( Supplementary Table 1 ). Primers flanking these loci were designed to yield 100- to 200-bp amplicons ( Supplementary Table 2 ). The relative quantity of loci present in anti-γH2AX immunoprecipitated chromatin from scratched versus confluent monolayers was expressed as a normalized ratio for each locus (qPCR results for six loci are shown in Fig. 4b,c ). Among the loci with known somatic mutations in GBM, the mean γH2AX ratio from four biological replicates was 1.25 (95% confidence interval (CI): 1.003–1.370) for the 135-bp window beginning at chr 13: 49,033,808 (GRCh37), located within exon 20 of Rb1 . Exon 20 contains several hotspots for recurrent mutations of high functional impact [37] . The other loci, including one located in exon 23 of Rb1 , had significantly lower mean γH2AX ratios, ranging from 0.72 to 1.01 ( Fig. 4d ). Among loci selected from genes exhibiting differential expression in scratched compared with confluent fetal NHAs, the 88-bp window beginning at chr 10: 70,847,873, located within exon 1 of Srgn had the highest mean γH2AX ratio (1.14, 95% CI: 1.01–1.28) ( Fig. 4e ). Srgn also demonstrated 33.9-fold higher expression in scratched fetal NHAs than in confluent NHAs and was the single, most overexpressed gene ( Supplementary Table 1 ). Mean normalized ratios of loci underexpressed in scratched NHAs ranged from 0.79 to 0.84, but none had an upper bound of the 95% CI<1. These results support the notion that scratch activation produces detectable changes in the pattern of γH2AX accumulation after IR in a gene locus-specific manner. Two loci, one in Rb1 and one in Srgn , which exhibited significantly elevated levels of γH2AX in the scratch state, were selected for further analysis. Detection of chromosomal rearrangements in Rb1 and Srgn Paired or multiple DSBs in close proximity may result in chromosome translocations, a key pathogenic event in the development of many solid and haematopoietic neoplasms [38] . To determine whether the higher levels of γH2AX at loci within Rb1 and Srgn in scratched versus confluent fetal NHAs after IR were associated with a higher frequency of chromosome breaks or rearrangements at those loci, we employed a strategy of inverse PCR [39] , [40] . Using SpeI and AarI restriction sites for Rb1 , and NheI and PacI restriction sites for Srgn ( Fig. 5a , Supplementary Fig. 15a , and Supplementary Table 3 ), we performed inverse PCR on scratched and confluent fetal and adult NHAs, both with and without 5 Gy of IR. This permitted the interrogation of a 6- to 9-kb region of interest for IR breakpoints and rearrangements. 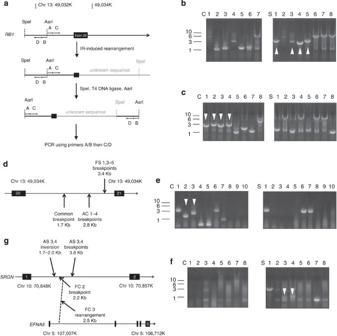Figure 5: Inverse PCR analysis ofRb1andSrgnfor transcriptional state-specific chromosomal breakpoints and rearrangements. (a) Schematic showing strategy for detection of chromosomal aberrations in the 6.2 kb region downstream ofRb1exon 20 using NheI and PacI. (b) Inverse PCR-amplifiedRb1products from aliquots (numbered) of irradiated confluent (C) or scratch (S) fetal NHA DNA were resolved on a 0.8% agarose gel. DNA ladder scale is in kb. Arrowheads indicate PCR products referred to ind. (c) Same as inb, except using adult NHA DNA. (d) Schematic showing relative locations of common, scratched fetal NHA (FS, products fromb, right) and confluent adult NHA (AC, products fromc, left) IR breakpoints. Genomic distances are relative toRb1exon 20. (e) Same as inbforSrgnusing fetal NHA DNA. Arrowheads indicate PCR products referred to ing. (f) Same as ine, except using adult NHA DNA. (g) Schematic showingSrgnchromosome rearrangments identified from confluent fetal (FC, products frome, left) and scratched adult (AS, products fromf, right) samples. Genomic distances are relative toSrgnexon 1. After IR, cells were allowed to repair DSBs for a period of 24 h. Figure 5: Inverse PCR analysis of Rb1 and Srgn for transcriptional state-specific chromosomal breakpoints and rearrangements. ( a ) Schematic showing strategy for detection of chromosomal aberrations in the 6.2 kb region downstream of Rb1 exon 20 using NheI and PacI. ( b ) Inverse PCR-amplified Rb1 products from aliquots (numbered) of irradiated confluent (C) or scratch (S) fetal NHA DNA were resolved on a 0.8% agarose gel. DNA ladder scale is in kb. Arrowheads indicate PCR products referred to in d . ( c ) Same as in b , except using adult NHA DNA. ( d ) Schematic showing relative locations of common, scratched fetal NHA (FS, products from b , right) and confluent adult NHA (AC, products from c , left) IR breakpoints. Genomic distances are relative to Rb1 exon 20. ( e ) Same as in b for Srgn using fetal NHA DNA. Arrowheads indicate PCR products referred to in g . ( f ) Same as in e , except using adult NHA DNA. ( g ) Schematic showing Srgn chromosome rearrangments identified from confluent fetal (FC, products from e , left) and scratched adult (AS, products from f , right) samples. Genomic distances are relative to Srgn exon 1. Full size image For Rb1 , DNA from irradiated scratched fetal NHAs demonstrated enrichment in inverse PCR products 2–3 kb in size compared with irradiated confluent NHAs ( Fig. 5b ). No such difference was seen when non-irradiated scratched and confluent fetal NHAs were compared ( Supplementary Fig. 15b ). Sequencing of the products revealed them to be the result of unrepaired DSBs 3.4 kb downstream of the coding region for exon 20, suggesting that this region is particularly susceptible to breakage in the scratch state. All conditions exhibited a breakpoint 1.7 kb downstream of exon 20 ( Fig. 5d ). The same analysis performed on adult NHAs revealed a breakpoint at 2.2 kb that was unique to the confluent state ( Fig. 5c,d and Supplementary Fig. 15c ). Inverse PCR analysis of the Srgn locus revealed amplification products unique to the irradiated confluent state in fetal NHAs ( Fig. 5e and Supplementary Fig. 15d ). One was identified as a rearrangement with chr 5: 106,994,943, located within intron 1 of Efna5 ( Supplementary Table 4 ). The other corresponded to a breakpoint present in the confluent but not scratch state ( Fig. 5g ). Analysis of irradiated scratched adult NHAs identified products containing an inversion of a segment of intron 1 and another product that harboured a partial deletion of intron 1 and a unique breakpoint ( Fig. 5f ). None of these products was observed in irradiated confluent adult NHAs or non-irradiated cells ( Supplementary Fig. 15d,e ). Taken together, these results indicate that the pattern of IR-induced DSBs and chromosome misrepair in NHAs is altered both by activation state and whether astrocytes are derived from a fetal or adult source. We demonstrate this phenomenon at two loci that were selected on the basis of high differential γH2AX activity in confluent and scratched fetal cells. Whole-genome distribution of γH2AX foci To examine differences in the pattern of IR-induced DSB repair in confluent and scratched NHAs genomewide, DNA from input and anti-γH2AX-immunoprecipitated chromatin was hybridized to whole-genome promoter arrays. In the confluent adult NHA samples, there was a characteristic distribution of γH2AX foci that was apparent in all three biological replicates ( Fig. 6a ). In particular, the small gene-dense chromosomes 16, 19, 20 and 22 exhibited higher-than-expected numbers of foci, whereas lower-than-expected numbers were observed in chromosomes 3, 6, 13 and X. In scratched adult NHA samples, this basic pattern was retained ( Fig. 6b and Supplementary Fig. 16a ), although the distribution, in general, appeared more random in nature (that is, observed-to-expected ratios closer to 1), possibly due to greater saturation of open chromatin domains by DSBs ( Fig. 3g , H3K4). 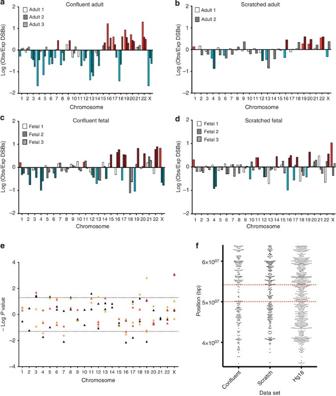Figure 6: Whole-genome distribution of γH2AX foci after IR. (a) Observed-to-expected ratio of foci after 5 Gy IR by chromosome in confluent adult NHAs. Coloured bars indicate that the difference between observed and expected numbers of foci was significant (P<0.05, Fisher’s exact test). (b–d) Same as inafor scratched adult, confluent fetal and scratched fetal NHAs, respectively. (e) Observed numbers of foci after IR are compared in confluent and scratched adult NHAs by genomic region using Fisher’s exact test. Negative log(P-values) indicate that scratched cells exhibited fewer foci than confluent cells at the specified significance level. Black, red and orange points indicate entire chromosome, short arm and long arm, respectively. Dashed lines indicateP=0.05. (f) Map of all γH2AX foci in confluent and scratched adult NHAs after 5 Gy IR (data from adults 1 and 2 combined) on the short arm of chromosome 19. A map of all 19q promoters present on the microarray is provided for reference. Region between dashed red lines exhibited significantly higher numbers of foci in the scratched compared with confluent state (P=0.0298, Fisher’s exact test). SeeSupplementary Table 3for identities of peaks in this region. Figure 6: Whole-genome distribution of γH2AX foci after IR. ( a ) Observed-to-expected ratio of foci after 5 Gy IR by chromosome in confluent adult NHAs. Coloured bars indicate that the difference between observed and expected numbers of foci was significant ( P <0.05, Fisher’s exact test). ( b – d ) Same as in a for scratched adult, confluent fetal and scratched fetal NHAs, respectively. ( e ) Observed numbers of foci after IR are compared in confluent and scratched adult NHAs by genomic region using Fisher’s exact test. Negative log( P -values) indicate that scratched cells exhibited fewer foci than confluent cells at the specified significance level. Black, red and orange points indicate entire chromosome, short arm and long arm, respectively. Dashed lines indicate P =0.05. ( f ) Map of all γH2AX foci in confluent and scratched adult NHAs after 5 Gy IR (data from adults 1 and 2 combined) on the short arm of chromosome 19. A map of all 19q promoters present on the microarray is provided for reference. Region between dashed red lines exhibited significantly higher numbers of foci in the scratched compared with confluent state ( P =0.0298, Fisher’s exact test). See Supplementary Table 3 for identities of peaks in this region. Full size image In the fetal NHA samples, where we also had three biological replicates available for analysis, higher-than-expected numbers were seen consistently in chromosomes 16 and 22 in both the confluent and scratched states. Chromosome 4, with particularly low gene density, demonstrated lower-than-expected numbers of foci in both states ( Fig. 6c,d ). Again, the overall distribution of foci appeared more random in the scratch compared with confluent state ( Supplementary Fig. 16b ). Using both H3K4me2/3 chrmatin immunoprecipitation (ChIP)–qPCR at selected loci ( Supplementary Fig. 17 ) and differential gene expression microarray data from confluent and scratched fetal NHAs ( Supplementary Fig. 18 ), we found a correlation between gene transcriptional activity and levels of γH2AX after irradiation. These results are consistent with our above observations that overall levels of H3K4me2/3 increase after scratch activation, and that H3K4me2/3 and γH2AX co-localize spatially within cell nuclei. To identify smaller genomic regions exhibiting significant changes in numbers of foci between the confluent and scratched states, we re-analysed the data by chromosome arm. In adult NHA samples, foci on chromosome arms 3p, 19q and Xp accounted for most of the increases in foci number seen on those chromosomes as a whole in the scratched state ( Fig. 6e ). The large number of foci observed on 19q allowed the identification of a smaller hotspot region, located between position 50 and 54 Mb (GRCh37), which contained significantly higher numbers of foci in the scratch compared with confluent state ( Fig. 6f and Supplementary Table 5 ). In fetal NHA samples, foci on chromosome arms 2q and Xq accounted for most of the increases in foci number seen on those chromosomes as a whole in the scratched state ( Supplementary Fig. 16c ). From these results we conclude that NHAs exhibit a characteristic genome-wide pattern of IR-induced DSB repair, and that this pattern is altered both by scratch activation and the developmental stage of the individual from which the NHAs are cultured. Furthermore, with a sufficient number of data points it is possible to identify smaller genomic regions that acquire large numbers of γH2AX foci in particular transcriptional states. Using complementary cellular, molecular and genomic approaches, we have shown that the transcriptional state of primary culture-derived human astrocytes directly has an impact on the pattern of DNA DSB repair and misrepair after exposure to IR. Previous investigations have demonstrated that activated neonatal mouse and rat astrocytes can be used to generate neurospheres [22] , [23] and are sensitized to neoplastic transformation after exposure to IR [41] , [42] . Furthermore, epidemiologic studies have established links between a variety of human malignancies and childhood exposure to ultraviolet and IR [43] , [44] , [45] . However, the mechanistic link between activation, differentiation state and oncogenesis is unclear. As DSBs are known to occur preferentially in open versus closed chromatin domains in a variety of cell types [32] , [33] , [34] , one possible unifying explanation is that changes in the transcriptional state of the cell shift loci between domains, thereby altering their susceptibility to breakage, spatial proximity to other susceptible loci and accessibility to DNA repair machinery. Sensitization to transformation may arise from a pro-neoplastic set of genomic alterations that occurs with greater probability in certain epigenetic states. In our experimental system, small structural variants and an interchromosomal fusion event were identified 24 h after irradiation of contact-inhibited NHAs, or actively migrating NHAs that had lost contact inhibition but had largely not entered S-phase ( Supplementary Fig. 7 ), implicating NHEJ as the most probable mechanism of DSB misrepair. In other phases of the cell cycle, it has recently been shown that homologous recombination is the predominant DSB repair mechanism near actively transcribed loci [46] . An area of future investigation will be to assess the relative contributions of homologous recombination, and more inherently error-prone pathways such as NHEJ, to genomic instability in pre-neoplastic and neoplastic cells. The differences we identified between fetal and adult NHAs in the genome-wide distribution of radiation-induced DSBs, DSB repair capacity and DSB misrepair patterns suggests that chromatin organization may play a significant role in determining a cell’s potential to undergo neoplastic transformation. This offers the possibility of new approaches to characterizing tumour initiating and maintaining cell populations, which complement traditional strategies that rely on gene expression patterns and cell surface markers.This work therefore provides a rationale and strategy for comparative mapping of genomic instability in cells of varying lineage and transcriptional state. Such explorations will enable investigators to trace observed chromosomal alterations in malignant solid neoplasms to misrepair events in potential cells of origin, and vice versa. The recurrent Srgn - Efna5 gene fusion we identified in irradiated confluent fetal NHAs warrants further investigation in malignant gliomas since both serglycin [47] and ephrin-A5 (ref. 48 ) are known to have functional significance in cancer. Moreover, the hotspot region of DSB repair in 19q (50–54 M) we identified in scratched adult NHAs harbours a number of genes implicated in oncogenesis, including Gltscr1 (ref. 49 ), Sympk [50] , [51] and notably Cic , in which loss of heterozygosity has recently been linked to the development of oligodendrogliomas [52] . Comparative mapping in the setting of histone deacetylase inhibitors, alkylating chemotherapies and targeted agents will also shed light on the contribution of treatment-induced chromosomal alterations to the development of therapeutic resistance. Tissue culture Fetal NHAs derived from second trimester cerebral cortex were purchased cryopreserved after first passage (ScienCell Research Laboratories). After thawing in a 37 °C water bath, 1 × 10 6 cells were plated on poly- L -lysine-coated 75-cm 2 polystyrene tissue culture flasks in human astrocyte medium containing 2% serum and astrocyte growth factors (ScienCell). Cells were grown to >90% confluence, trypsinized (trypsin-EDTA 0.5% w/v, Invitrogen) and replated for experiments. Adult NHAs were obtained from frontal or temporal lobe neocortex excised during cortical resections for epilepsy. Directly adjacent histological sections were reviewed by a neuropathologist and confirmed to exhibit minimal gliosis and no evidence of dysplasia. Cultures were initiated as previously described [53] , [54] , with modifications briefly described as follows. Fresh cortical specimens were placed on wet ice and washed in PBS containing 2% penicillin–streptomycin–neomycin mixture (Invitrogen) and 1% antifungal solution (Fungizone, Invitrogen). Grey matter was isolated using a scalpel, minced finely and digested in 20 ml 0.5% w/v trypsin-EDTA for 20 min at 37 °C. Bovine pancreatic DNase I (400 U, Sigma) was added and the tissue was incubated for an additional 10 min. After centrifugation at 500 g for 5 min, cells at the top of the pellet were plated on uncoated 75-cm 2 tissue culture flasks for 2 h in complete astrocyte medium, to allow monocytes and macrophages to adhere. The supernatant was then replated on poly- L -lysine-coated 75-cm 2 tissue culture flasks. The medium was changed after 48 h and then every 4 days until adherent cells achieved confluence. Simian astrocytes were obtained from necropsy specimens of adult Macaca fascicularis temporal lobe within 1 h of animal euthanization as previously described [55] . Briefly, grey matter was isolated, disaggregated and enzymatically digested for 30 min. Cells were plated in uncoated flasks in medium containing RPMI 1640, 2 mM glutamine, 1% penicillin–streptomycin–neomycin mixture, 0.5% antifungal solution and 10% fetal bovine serum. Incubation for 1 h at room temperature with L -leucine methyl ester (10 mM) was used to remove microglia and macrophages. The medium was changed every 4 days, after vigorous shaking to remove neurons and oligodendrocytes, until adherent cells achieved confluence. The NINDS/NIDCD Animal Care and Use Committee and NIH Clinical Center Institutional Review Board approved all animal and tissue procurement protocols. Informed consent was obtained from human subjects donating tissue. Scratching of monolayers Monolayers of astrocytes allowed to grow to 100% confluence over a period of 10–14 days were scratched using a sterile pipette tip. For proliferation experiments, monolayers in six-well plates were scratched with a 200-μl pipette tip in a 4 × 4 grid pattern. For immunofluorescence experiments, monolayers in chamber slides were scratched once linearly with a 200-μl pipette tip. For gene expression and ChIP experiments, monolayers in 15-cm diameter petri dishes were scratched with a 10-ml pipette tip in a 7 × 7 grid pattern. For inverse PCR experiments, monolayers in 10-cm diameter petri dishes were scratched with 1,000 μl pipette tip in a 5 × 5 grid pattern. In all cases, the culture medium was changed immediately after scratching to remove non-adherent cells. Irradiation Cells were irradiated in an X-ray irradiator (X-RAD 320, Precision X-ray Inc.) at room temperature in ambient air. A dose of 5 Gy was administered over 2 min. Cells were transferred back to a 37 °C incubator within 10 min of irradiation. Immunofluorescence Cells in chamber slides were fixed with Histochoice fixative solution (Mandel) for 10 min after three gentle washes in PBS to remove media. Cells were washed again with PBS, permeabilized with PBS containing 0.03% Triton-X for 20 min and then blocked (Superblock in PBS, Thermo) overnight at 4 °C. The following primary antibodies, diluted in blocking solution, were applied and incubated for 12 h at 4 °C: mouse anti-GFAP (1:500; Cell Signaling, 3670), rabbit anti-GFAP (1:500; Invitrogen, 18-0063), mouse anti-nestin (1:200; Santa Cruz, sc-71665), mouse anti-SOX2 (1:100; Cell Signaling; 4900), mouse anti-γH2AX (1:200; BD Pharmingen, 560443), rabbit anti-γH2AX (1:200; Cell Signaling, 9718), rabbit anti-H2AX (1:200; Cell Signaling, 7631), rabbit anti-H2AX (1:500; Cell Signaling, 2595), mouse anti-H3K4Me2/3 (1:200; Abcam, ab6000), rabbit anti-H3K4Me2/3 (1:200; Cell Signaling, 9727), mouse anti-H3K9Me2/3 (1:100; Cell Signaling, 5327), mouse anti-53BP1 (1:500; Upstate, NY, 05-726). Cells were washed with PBS three times to remove primary antibodies and the following secondary antibodies were applied for 2 h in the dark at room temperature: Alexa Fluor 488 donkey anti-mouse IgG (1:500; Invitrogen, A21202), Alexa Fluor 555 donkey anti-rabbit IgG (1:500; Invitrogen, A31572). Cells were counterstained with Hoescht or 4′,6-diamidino-2-phenylindole for 20 min and mounted (Vectashield Hard Set, Vector Laboratories) for confocal microscopy. All immunofluorescence imaging was performed on a Zeiss LSM 510 confocal laser scanning microscope using the manufacturer’s software. Western blot analysis Protein was extracted from NHA cell pellets using RIPA lysis buffer supplemented with Halt proteinase inhibitor cocktail (Thermo). After vortexing and centrifugation at 12,000 g for 10 min at 4 °C, supernatant was collected and protein was quantified using a Bio-Rad protein assay kit (Hercules, CA, USA). Equal amounts of protein for each sample were separated on a NuPAGE 4–12% Bis-Tris gel (Invitrogen) and transferred to polyvinylidene difluoride membranes (Invitrogen). Membranes were blocked in Blocking Buffer (Invitrogen) at 4 °C overnight before application of primary antibodies. The following primary antibodies were used: γH2AX, H3K4Me2/3, H3K9Me2/3, SOX2, nestin (1:1,000; manufacturers as above); H2AX (1:400; Cell Signaling, 2595); Rpb1 (1:1,200; Cell Signaling, 2629); β-actin (1:1,000; Santa Cruz Biotechnology, sc-130301). Horseradish peroxidase-conjugated anti-mouse or anti-rabbit secondary antibody (1:5,000; Santa Cruz Biotechnology, sc-2004 and sc2005) was applied for 1 h at room temperature. Blottings were visualized using chemiluminescence (Thermo). Immunoprecipitated chromatin samples were eluted from protein G magnetic beads, reduced and resolved on 4–12% NuPAGE Novex Bis-Tris gels (Invitrogen), according to the manufacturer’s protocol. Samples were then transferred to polyvinylidene difluoride membranes, blocked with 5% skim milk and blotted with rabbit anti-γH2AX monoclonal antibodies (1:1,000; Cell Signaling, 9718). Proteins were detected by chemiluminescence. Proliferation assays To determine the proliferation capacity of adherent cells following treatment with scratch and/or irradiation, cells were trypsinized from a single well in a six-well plate and counted with a hemocytometer using trypan blue. The cells in each treatment group, along with controls, were plated on coated 25-cm 2 tissue culture flasks in human astrocyte medium containing 2% serum and astrocyte growth factors (ScienCell) at a density of 3,000 cells per cm 2 and allowed to grow to 70%–90% confluence, at which point the cells were trypsinized, counted and reseeded in flasks at a density of 3,000 cells per cm 2 . Numbers of cells obtained at each passage were used to track the PDL over time, where ΔPDL=log 2 [(number of cells obtained at passage)/(number of cells seeded)]. Chromatin immunoprecipitation Astrocytes were grown in 15-cm culture dishes and chromatin was cross-linked with 1% formaldehyde. At least 1 × 10 7 fetal NHAs and 2 × 10 6 adult NHAs were used for each condition. Immunoprecipitation of nuclease S7-digested chromatin was performed using the SimpleChIP kit with protein G magnetic beads (Cell Signaling), according to the manufacturer’s protocol. The following ChIP-grade antibodies were used: rabbit anti-histone H3 (1:50; Cell Signaling, 4620), normal rabbit IgG (1:200; Cell Signaling, 2729), rabbit anti-γH2AX (1:100; Abcam, ab2893), mouse anti-H3K4me2/3 (1:100; Cell Signaling, 9727). Quantitative PCR For each pair of forward and reverse primers ( Supplementary Table 2 ), SYBR green assays (Applied Biosystems) were used to quantify the amount of genomic DNA precipitated using anti-γH2AX antibodies relative to input DNA samples. Results were normalized to positive control samples precipitated using anti-histone H3 antibodies after subtracting out signal due to normal rabbit IgG-precipitated negative controls. Serially diluted input samples were used to determine the efficiency of the reaction for each primer set each time an assay was performed. The normalized signal from scratched samples was divided by the corresponding signal from control samples to determine the normalized γH2AX ratios indicated in Fig. 4d,e . All assays were performed with two technical and at least four biological replicates. Inverse PCR Genomic DNA from each experimental condition (confluent, scratched, irradiated, scratched and then irradiated) was purified from at least 1 × 10 6 cells using the Nucleospin Tissue kit (Macherey-Nagel), according to the manufacturer’s protocol. RNA was removed by incubating with RNase A (10 mg ml −1 ) at room temperature for 5 min. Five hundred nanograms of purified DNA was used for each restriction digest. Restriction enzymes (New England BioLabs) and conditions used were as follows: NheI, 10 units incubated at 37 °C for 60 min in a total volume of 50 μl 1 × NEBuffer 2 supplemented with 10 μg ml −1 BSA; PacI, 10 units incubated at 37 °C for 60 min in a total volume of 50 μl NEBuffer 1 supplemented with 10 μg ml −1 BSA; KpnI, 10 units incubated at 37 °C for 60 min in a total volume of 50 μl 1 × NEBuffer 1 supplemented with 10 μg ml −1 BSA; BsaWI, 10 units incubated at 60 °C for 60 min in a total volume of 50 μl 1 × NEBuffer 4 supplemented with 10 μg ml −1 BSA; T4 DNA ligase, 1,200 units incubated at 20 °C for 30 min in a total volume of 40 μl 1 × NEBuffer T4 supplemented with 1 mM ATP. Between and after digests, DNA was repurified in water using spin columns (Qiaquick, Qiagen). Purified digested DNA was divided into aliquots of 50 ng and amplified using primers A/B and fully nested primers C/D ( Fig. 5a , Supplementary Fig. 15a and Supplementary Table 4 ) in a long-range PCR reaction (Qiagen LongRange, Qiagen or KlenTaq LA DNA Polymerase Mix, Sigma) on a thermal cycler (Eppendorf Mastercycler) in a reaction volume of 50 μl. An annealing temperature of 65 °C, extension time of 8 min at 68 °C and 35 cycles provided adequate results for both Rb1 and Srgn . Before amplification using nested primers, PCR products were incubated with 2 units of Klenow fragment supplemented with 33 μM each dNTP for 15 min at 25 °C to blunt ends, then purified in a spin column. DNA sequencing and alignment Inverse PCR products were purified in water using Qiaquick spin columns (Qiagen). Sufficient amounts (up to 100 ng, depending on size of product) were combined with 3.2 pmol of sequencing primer and provided to the NINDS DNA Sequencing Core Facility for BigDye Terminator sequencing on an ABI 3130 genetic analyser (Applied Biosystems). Chromatograms were manually checked for integrity and sequences were aligned to human genome build GRCh37.3 (NCBI) using the blastn algorithm ( http://blast.ncbi.nlm.nih.gov ). ChIP-chip Input and anti-γH2AX immunoprecipitated chromatin was uncross-linked and genomic DNA was purified using DNA spin columns (Qiaquick, Qiagen). Samples were amplified using the GenomePlex Complete Whole Genome Amplification kit (Sigma) without further fragmentation, to obtain sufficient quantities of DNA (>2 μg) for labelling and microarray hybridization. Input and confluent or scratched samples were co-hybridized to human 385 K RefSeq Promoter arrays (Roche Nimblegen), according to the manufacturer’s protocol, and analysed using DEVA v1.2.1 software. Peaks were mapped to human genome build GRCh36.1 (NCBI) and verified in build GRCh37.3. The expected number of DSBs for a given genomic region was determined by dividing the number of promoters in the region by the total number of promoters represented on the chip, then multiplying by the total number of peaks observed at a false discovery rate of 0.20. The ratio of observed-to-expected number of peaks was then plotted by chromosome and analysed using Fisher’s exact test. Neutral comet assay Fetal NHAs were grown to 100% confluence in each well of a six-well tissue culture plate over 10 days. Two wells were scratched with a 1,000-μl pipette tip, each well was washed three times with PBS and the medium was changed in all wells. Twenty four hours later, cells were irradiated with 5 Gy of X-rays over a period of 2 min and then returned to a 37 °C incubator. At the specified time points, cells were trypsinized, resuspended at a concentration of 1 × 10 5 cells per ml of ice-cold PBS and then mixed at a 1:10 ratio (v/v) with low-melting-point agarose (Trevigen). Cell suspensions were placed on slides and agarose was allowed to cool for 30 min at 4 °C in the dark. Slides were then lysed for 1 h at 4 °C in the dark in pre-chilled lysis buffer. Slides were washed with cold tris-borate-EDTA electrophoresis solution and placed in a horizontal electrophoresis chamber. A voltage of 22 V (1.0 V cm −1 ) was applied for 10 min. Slides were dehydrated in 70% ethanol for 5 min and were allowed to air dry overnight in the dark. Samples were then stained with propidium iodide, coverslipped and visualized immediately. Comets were visualized with a fluorescence microscope and images were analysed using freely available CASPlab software ( www.casplab.com ). BrDU pulse assay NHAs were grown to 100% confluence on glass chamber slides over 10–14 days and then linearly scratched with a 200-μl pipette tip. Medium was removed and replaced with medium containing 10 μM BrDU (Sigma). After 30 min to 24 h, medium was removed, cells were washed with PBS and medium not containing BrDU was reapplied. At 24 h, cells were fixed for 10 min with Histochoice (Mandel), washed three times with PBS and denatured with 2 M HCl at 37 °C for 1 h. HCl was neutralized with three washes of tris-borate-EDTA buffer. Cells were then permeabilized for 20 min with PBS containing 0.03% Triton-X and blocked with Superblock in PBS (Thermo) for 90 min at 37 °C. Mouse anti-BrDU primary antibodies were applied (1:200, BD Pharmingen, 555627) for 12 h at 4 °C. After three washes with PBS, Alexa Fluor 488 donkey anti-mouse secondary antibodies (1:500; Invitrogen, A21202) were applied for 2 h in the dark at room temperature and slides were prepared for confocal microscopy as described in Methods. α-Amanitin treatment Fetal NHAs were grown to 100% confluence on 10 cm poly- L -lysine-coated Petri dishes over 7–10 days and then scratched in a 5 × 5 grid pattern with a 10-ml pipette tip. The medium in each dish was changed and the cells at the scratch edges allowed to migrate at 37 °C in an incubator. For α-amanitin conditions, α-amanitin containing medium (10 or 50 μg ml −1 ) was applied to the dishes after 24 h of migration and incubated for 24 h. Cells were then irradiated (5 Gy) and, after 30 min, were prepared for western blotting as described above. Pretreatment, sham treatment and non-scratched monolayers were used as controls. Gene expression analysis Total RNA was isolated from 1 × 10 6 confluent and scratched fetal NHAs using RNeasy Micro kits (Qiagen), amplified using Arcturus RiboAMP kits (Applied Biosystems), labelled using Cy5-dUTP or Cy3-dUTP as described previously [56] and hybridized to ROSP human 8 K complementary DNA oligo-arrays (NCI, GEO platform GPL6665). Hybridized arrays were scanned using a GenePix 4000A scanner (Axon Instruments) and images were analysed with GenePix Pro 4.0 software (Axon Instruments). Raw signal intensities were normalized using standard LOESS method and log2 transformed for further analysis in SAM 4.0 (Stanford University). Additional replicate data for confluent and scratched fetal NHAs was generated using Affymetrix Human Gene 1.0 ST arrays in the NHGRI intramural microarray core facility. How to cite this article: Yong, R. L. et al. Cell transcriptional state alters genomic patterns of DNA double-strand break repair in human astrocytes. Nat. Commun. 5:5799 doi: 10.1038/ncomms6799 (2014). Accession codes: All gene expression data have been deposited in the NCBI Gene Expression Omnibus under accession code GSE45994 .